Biological interpretation of genome-wide association studies using predicted gene functions The main challenge for gaining biological insights from genetic associations is identifying which genes and pathways explain the associations. Here we present DEPICT, an integrative tool that employs predicted gene functions to systematically prioritize the most likely causal genes at associated loci, highlight enriched pathways and identify tissues/cell types where genes from associated loci are highly expressed. DEPICT is not limited to genes with established functions and prioritizes relevant gene sets for many phenotypes. The causal variants, genes and pathways in many genome-wide association studies (GWAS) loci often remain elusive, due to linkage disequilibrium (LD) between associated variants, long-range regulation and incomplete biological knowledge of gene function. To translate genetic associations into biological insight, we need at a minimum to identify the genes that account for associations as well as the pathways and tissue/cell type context(s) in which the genes’ actions affect phenotypes. Although cell-type-specific expression quantitative trait loci (eQTLs) or coding (non-synonymous) variants in strong LD with associated variants can potentially link these variants to genes, overlap with eQTLs or coding variants may be coincidental. In addition, coding variants in high LD with associated variants are rarely observed, and eQTL data from non-haematological cell types are rare. Direct functional follow-up of the many potentially causal variants and genes is typically difficult and expensive, so an attractive first step is to use computational approaches to prioritize genes in associated loci with respect to their likely biological relevance, and to identify pathways and tissues to define their likely biological context. The current paradigm for gene prioritization methods is to systematically search for commonalities in functional annotations between genes from different associated loci, such as shared features derived from text mining [1] (which is limited by the literature’s highly incomplete characterization of gene function) or propensity to interact at the protein level [2] (which is unlikely to capture the full functional spectrum of a given gene or phenotype [3] ). The paradigm for gene set analysis is to search for enrichment of the genes near associated variants in manually curated gene sets or in gene sets derived from molecular evidence [4] . Although certain pathways have been carefully characterized, and manually curated gene sets and protein–protein interaction maps can be of great value, pathway annotation of genes remains sparse and skewed towards well-studied genes [5] . At the same time, the availability of large, diverse, genome-wide data sets, such as gene expression data, can elucidate and annotate potential functional connections between genes [6] . Given these limitations and opportunities, and the wide spectrum of traits and diseases analysed in association studies, there is a need for a general computational approach that integrates diverse, non-hypothesis-driven data sets to prioritize genes and pathways [7] , [8] . With the goal of meeting this need, we develop and hereby present a framework called Data-driven Expression Prioritized Integration for Complex Traits (DEPICT, www.broadinstitute.org/depict ), which is not driven by phenotype-specific hypotheses and considers multiple lines of complementary evidence to accomplish gene prioritization, pathway analysis and tissue/cell type enrichment analysis. This framework can prioritize genes, pathways and tissue/cell types across many different phenotypes [9] , [10] , [11] , [12] , [13] . Overview of the DEPICT methodology DEPICT builds on our recent work that used co-regulation of gene expression (derived from expression data of 77,840 samples), in conjunction with previously annotated gene sets, to accurately predict gene function based on a ‘guilt-by-association’ procedure [6] . We first expanded this approach to include 14,461 existing gene sets, representing a wide spectrum of biological annotations (including manually curated pathways [14] , [15] , [16] , molecular pathways from protein–protein interaction screens [17] and phenotypic gene sets from mouse gene knock-out studies [18] ). By calculating, for each gene, the likelihood of membership in each gene set (based on similarities across the expression data; see Methods), we generated 14,461 ‘reconstituted’ gene sets (see Fig. 1 ; Supplementary Data 1 ). Rather than traditional binary gene sets (genes are included or not included), these reconstituted gene sets contain a membership probability for each gene in the genome; conversely, a gene is functionally characterized by its membership probabilities across the 14,461 reconstituted gene sets. Using these precomputed gene functions and a set of trait-associated loci, DEPICT assesses whether any of the 14,461 reconstituted gene sets are significantly enriched for genes in the associated loci, and prioritizes genes that share predicted functions with genes from the other associated loci more often than expected by chance. In addition, DEPICT utilizes a set of 37,427 human microarrays to identify tissue/cell types in which genes from associated loci are highly expressed. DEPICT uses precomputed GWAS based on randomly distributed phenotypes to take sources of confounding into account: it extracts gene-density-matched input loci from these ‘null GWAS’, recomputes results and adjusts the P values from the above three analyses for null expectation. It also uses the null GWAS to adjust for multiple testing by computing false discovery rates (FDRs, see Methods). 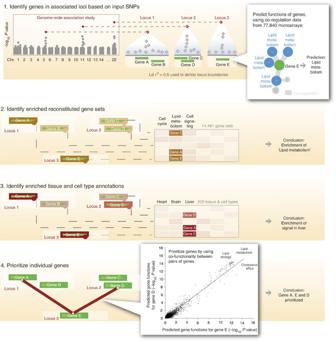Figure 1: Overview of DEPICT. DEPICT is designed to identify likely causal genes, functional or phenotypic gene sets that are enriched in genes within associated loci, and tissues or cell types that are implicated by the associated loci. DEPICT takes as input a set of trait-associated SNPs and uses them to identify independently associated loci that may comprise up to several genes. DEPICT uses co-regulation data from 77,840 microarrays to predict genes’ biological functions across 14,461 gene sets representing a wide spectrum of biological annotations and to construct 14,461 ‘reconstituted’ gene sets. DEPICT then uses this information to identify reconstituted gene sets that enrich for genes in the associated loci, and to prioritize genes at associated loci, by identifying genes in different loci that have similar predicted functions. Finally, DEPICT relies on 37,427 human gene expression microarrays to assess whether genes in associated loci are highly expressed in any of 209 tissue/cell type annotations. Figure 1: Overview of DEPICT. DEPICT is designed to identify likely causal genes, functional or phenotypic gene sets that are enriched in genes within associated loci, and tissues or cell types that are implicated by the associated loci. DEPICT takes as input a set of trait-associated SNPs and uses them to identify independently associated loci that may comprise up to several genes. DEPICT uses co-regulation data from 77,840 microarrays to predict genes’ biological functions across 14,461 gene sets representing a wide spectrum of biological annotations and to construct 14,461 ‘reconstituted’ gene sets. DEPICT then uses this information to identify reconstituted gene sets that enrich for genes in the associated loci, and to prioritize genes at associated loci, by identifying genes in different loci that have similar predicted functions. Finally, DEPICT relies on 37,427 human gene expression microarrays to assess whether genes in associated loci are highly expressed in any of 209 tissue/cell type annotations. Full size image Calibration of locus definitions Having developed this framework, we first considered a key feature, the definition of an associated locus—that is, given an associated variant, how many of the nearby genes should be taken into consideration as potentially causal? Using as a positive control Mendelian disease genes that affect skeletal growth and are over-represented in height-associated GWAS loci [10] , [19] , we evaluated DEPICT’s performance using loci defined by different combinations of genetic and physical distance from the lead associated variant ( Supplementary Data 2 ). We found that a locus definition of r 2 >0.5 from the lead variant was optimal ( Supplementary Note 1 ). We repeated the analysis using genome-wide-significant associations for low-density lipoprotein (LDL) cholesterol [20] and 14 Mendelian lipid genes [20] as positive controls and observed similar results ( r 2 >0.4), indicating that the calibration does not change drastically for other traits ( Supplementary Data 3 ). Type-1 error rate analysis We next tested whether DEPICT properly controls the type-1 error rate. Running DEPICT with random input loci based on either real genotype or simulated genotype data, we observed nearly uniform distributions for gene set enrichment, gene prioritization and tissue/cell type enrichment P values (see Supplementary Fig. 1 and Methods). Importantly, we did not observe any correlation between gene length and gene prioritization P values (Spearman r 2 =7.70 × 10 −5 ), nor correlation with locus gene density (Spearman r 2 =7.53 × 10 −8 ), two factors that have often confounded pathway analyses [21] . We also did not observe any correlation between tissue/cell type enrichment P values and the number of samples available in the expression data sets for each annotation (Spearman r 2 =6.9 × 10 −4 ), nor were results dependent on the particular set of genotype data used to construct the null GWAS ( Supplementary Note 2 ). Together, these results indicated that DEPICT results are not driven by bias in its data sources. Benchmarking the gene set enrichment framework We next compared DEPICT with two GWAS pathway methods, MAGENTA [22] and GRAIL [1] using GWAS results for three phenotypes, each with >50 independent genome-wide significant single-nucleotide polymorphisms (SNPs): Crohn’s disease [23] , human height [10] and LDL [20] . DEPICT’s gene set enrichment functionality outperformed MAGENTA (a widely used GWAS gene set enrichment tool) by identifying more relevant gene sets (both methods exhibited comparable type-1 error rates; Supplementary Figs 1 and 2 ) for all three phenotypes: DEPICT identified 2.5 times as many significant gene sets (FDR<0.05) for Crohn’s disease, 2.8 times as many significant gene sets for height and 1.1 times as many significant gene sets for LDL ( Fig. 2 ; Supplementary Figs 3–5 ; Supplementary Data 4–6 ). Many gene sets prioritized by DEPICT, but not MAGENTA, appear biologically relevant (for example, regulation of immune response, response to cytokine stimulus and toll-like receptor signalling pathway for Crohn’s disease; Fig. 2 ). To test whether our gene set reconstitution strategy was driving the performance differences between MAGENTA and DEPICT, we ran MAGENTA with non-probabilistic, binary (yes/no) versions of the reconstituted gene sets (see Methods). We found a consistent increase in the number of nominally significant gene sets when MAGENTA was run with reconstituted gene sets for Crohn’s disease, height and LDL (1.4, 1.6 and 1.7-fold increases, respectively, in number of nominally significant gene sets using the 95 percentile model; Supplementary Data 4–6 ; Supplementary Figs 6–8 ). To assess whether the reconstituted gene sets enhance the performance of DEPICT, we ran DEPICT using the original, predefined gene sets. As expected, the number of prioritized gene sets (FDR<0.05) dropped to 97.7, 92.9 and 20% for the Crohn’s disease, height and LDL analyses, respectively ( Supplementary Data 4–6 ). Together, these analysis indicate that the gene set reconstitution, combined with DEPICT’s ability to use probabilistic gene sets, is responsible for the increased performance of DEPICT compared with MAGENTA in gene set enrichment analysis. 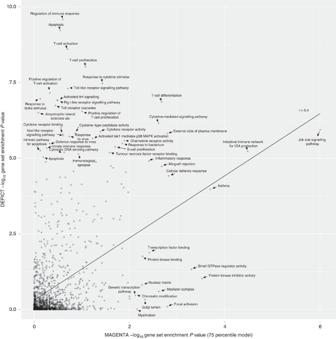Figure 2: Comparison of DEPICT and MAGENTA for Crohn’s disease. Comparison of DEPICT, which was run with 63 genome-wide significant Crohn’s disease SNPs as input, and MAGENTA, which was run using the complete list of Crohn’s disease summary statistics23(downloaded fromwww.ibdgenetics.org). DEPICT was run using 1,280 reconstituted gene sets, and MAGENTA was run using the predefined versions of the same 1,280 gene sets. Both methods were run with default settings and non-adjusted enrichmentPvalues are plotted. Figure 2: Comparison of DEPICT and MAGENTA for Crohn’s disease. Comparison of DEPICT, which was run with 63 genome-wide significant Crohn’s disease SNPs as input, and MAGENTA, which was run using the complete list of Crohn’s disease summary statistics [23] (downloaded from www.ibdgenetics.org ). DEPICT was run using 1,280 reconstituted gene sets, and MAGENTA was run using the predefined versions of the same 1,280 gene sets. Both methods were run with default settings and non-adjusted enrichment P values are plotted. Full size image Benchmarking the gene prioritization framework Using gene lists from whole-blood expression quantitative locus data [24] , rodent growth plate differential expression data [25] and Mendelian human lipid genes reported in literature [20] (see Methods), we constructed positive sets of genes to compare DEPICT’s gene prioritization performance with GRAIL (a widely used GWAS gene prioritization tool). DEPICT and GRAIL performed similarly in analyses based on all genome-wide significant loci with at least one positive gene, based on area under a receiver-operating characteristic (ROC) curve (AUC, Table 1 ; Supplementary Datas 7–9 ; Supplementary Fig. 9 ). However, when restricting the height comparison with loci with no well-known Mendelian human skeletal growth gene, DEPICT markedly outperformed GRAIL, prioritizing genes at many more loci (DEPICT: 1.1 genes per locus, GRAIL: 0.4 genes per locus), suggesting that DEPICT performs better at loci harbouring genes with less well-established roles in literature ( Supplementary Data 10 ). We validated this observation using genes nearest to height-associated SNPs as positive genes at these loci. The nearest gene is an unbiased, but highly imperfect benchmark (for example, only 13/21 Mendelian skeletal growth genes in a large height GWAS [19] were the nearest genes to a height-associated SNP), so AUC is expected to be low using this benchmark. Nonetheless, DEPICT not only prioritized more genes than GRAIL, but also had a higher AUC ( Supplementary Data 11 ). Finally, DEPICT performed consistently better than a gene expression-based version of GRAIL ( Supplementary Data 7–9 ), indicating that use of gene expression data in the prediction is not driving DEPICT’s superior performance across several of the comparisons. Together, these analyses indicate that DEPICT performs particularly well for gene prioritization at what are arguably the most important loci for new discovery: those with biology that is less well captured in already published literature. Table 1 Overview of DEPICT and GRAIL comparison. Full size table Prioritization of genes outside genome-wide significant loci We hypothesized that DEPICT could also be used to prioritize genes outside genome-wide significant loci, based on predicted functional relatedness to genes within genome-wide significant loci. Similar to the gene prioritization implemented in DEPICT, we prioritized genes with higher than expected pairwise similarities to genes from trait-associated loci (across the 14,461 functional predictions; see Methods). SNPs within or near (±50 kb) the 3,022 genes that were functionally related to Crohn’s disease loci genes (at FDR<0.05) had lower association P values than SNPs in the same number of unrelated genes (genes with FDR>0.99; genomic inflation factor λ =1.49 versus λ =1.31), indicating that DEPICT enriches for as-yet-unidentified genes associated with Crohn’s disease. The enrichment was further increased when considering only SNPs that overlap with eQTLs in whole blood [24] ( λ =1.69 versus λ =1.25). A similar enrichment of associations was seen for height ( λ =1.92 versus λ =1.62) and LDL ( λ =1.06 versus λ =0.97). To begin to assess the performance and specificity of DEPICT across a wider range of phenotypes, we applied DEPICT to 61 phenotypes in the NHGRI GWAS Catalog [26] that had at least 10 genome-wide-significant (unadjusted association P value<5 × 10 −8 ) associations. DEPICT identified at least one significantly enriched ( P value <10 −6 , the Bonferroni-corrected significance threshold) reconstituted gene set for 39 of the 61 phenotypes ( Fig. 3 ; Supplementary Data 12 ). To test whether DEPICT identified similar gene sets for related phenotypes, we clustered the 39 traits based on their gene set enrichment scores across the 14,461 reconstituted gene sets ( Fig. 3 ). Related traits clustered with each other, but different phenotypes yielded quite different gene sets. Furthermore, many of the top gene sets were of clear relevance to the phenotype ( Supplementary Data 12 ). Thus, DEPICT is able to identify, with specificity, biologically relevant gene sets for a wide range of human traits and diseases. Consistent with these results, we recently used DEPICT to analyse GWAS data for height, body mass index and waist–hip ratio adjusted for body mass index (from the GIANT Consortium) [10] , [12] , [13] and for hypospadias [9] . For each phenotype, DEPICT highlighted a distinct and biologically meaningful group of known and novel genes, gene sets and tissue/cell types. 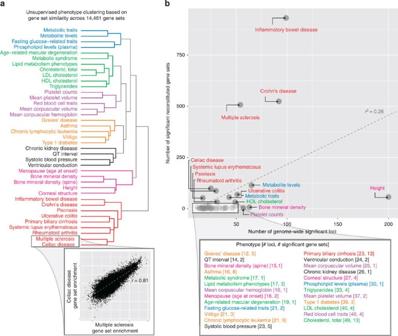Figure 3: DEPICT analysis using GWAS Catalog results. DEPICT identified at least one significant reconstituted gene set for 39 traits and diseases from the GWAS Catalog (we investigated 61 traits with at least 10 independent genome-wide significant loci). (a) Unsupervised clustering of the 39 phenotypes based on their gene set enrichment scores across all reconstituted gene sets yielded 7 clusters of phenotypes (roughly corresponding to metabolic, lipids, haematological, autoimmune, blood pressure/cardiac conduction, growth/bone/menopause and a second autoimmune cluster), which indicates that DEPICT is able to identify phenotypic-specific and biologically relevant gene sets for a wide range of phenotypes. The inset shows that the multiple sclerosis and coeliac disease gene set enrichment scores are highly correlated and therefore were clustered within the same clade. (b) The number of genome-wide significant loci for a given phenotype was positive correlated with the number of significant (FDR<0.05) reconstituted gene sets for that phenotype (Pearsonr2=0.26,t-testPvalue=6.86 × 10−5). Figure 3: DEPICT analysis using GWAS Catalog results. DEPICT identified at least one significant reconstituted gene set for 39 traits and diseases from the GWAS Catalog (we investigated 61 traits with at least 10 independent genome-wide significant loci). ( a ) Unsupervised clustering of the 39 phenotypes based on their gene set enrichment scores across all reconstituted gene sets yielded 7 clusters of phenotypes (roughly corresponding to metabolic, lipids, haematological, autoimmune, blood pressure/cardiac conduction, growth/bone/menopause and a second autoimmune cluster), which indicates that DEPICT is able to identify phenotypic-specific and biologically relevant gene sets for a wide range of phenotypes. The inset shows that the multiple sclerosis and coeliac disease gene set enrichment scores are highly correlated and therefore were clustered within the same clade. ( b ) The number of genome-wide significant loci for a given phenotype was positive correlated with the number of significant (FDR<0.05) reconstituted gene sets for that phenotype (Pearson r 2 =0.26, t -test P value=6.86 × 10 −5 ). Full size image We present a computational framework called DEPICT, which enables gene prioritization, gene set enrichment analysis and tissue/cell type enrichment analysis to generate specific testable hypotheses that are critical to inform experimental follow-up of GWAS. DEPICT implements these three distinct functionalities into a single, publicly available tool. Apart from providing useful insights into pathways and biological annotations of relevance to a phenotype, a key application of the gene set enrichment functionality is to use it for selecting in vitro phenotypes that may serve as readouts in cellular assays used to validate prioritized genes for a complex trait. A key advantage of DEPICT over existing tools is the gene set reconstitution, which enables prioritization of previously poorly annotated genes, as well as more specific and powerful gene set enrichment analysis. By using data sets and methods that are not specific to any particular disease or trait, DEPICT does not depend on phenotype-specific hypotheses (for example, particular neuronal gene sets being important for schizophrenia). On the basis of our current experience, we recommend employing DEPICT on genome-wide significant loci as well as all loci with association P values <10 −5 (see Supplementary Fig. 10 for results based on LDL loci using the relaxed threshold and for an example on visualizing DEPICT results). We also recommend a locus definition of r 2 >0.5 from lead SNPs. It is important to note that reconstituted gene sets should be interpreted in light of the genes that are mapped to them, rather than strictly by their identifiers (which are carried over from the predefined gene sets). Despite DEPICT’s ability to identify relevant gene sets for a large number of traits and diseases, the method may be less sensitive to phenotypes caused by genes that have specialized functions that cannot be well predicted based on integrating gene expression data with the currently existing predefined gene sets. Indeed, there are multiple ways in which the DEPICT framework could be improved further. Additional future work includes iteratively conditioning on significant genes, gene sets and tissue/cell types to enhance prioritization of genes with weaker, yet significant, relationships, and quantification of the relative importance of significant predictions. Additional expression data would enhance the data sources available for DEPICT, especially for prioritization of tissues/cell types. Other data types, such as epigenetic data, have yet to be integrated into the DEPICT framework, and DEPICT does not yet use information that could further prioritize genes within loci, such as LD with eQTLs or missense variation, or being the nearest gene to the lead SNP. Finally, DEPICT is currently optimized for GWAS results, but could be adapted to other types of data sets (custom arrays, exome chip or sequencing). In conclusion, there is a need for approaches that are not driven by phenotype-specific hypotheses and that consider multiple lines of complementary evidence to accomplish gene prioritization, pathway analysis and tissue/cell type enrichment analysis. We have developed a computational and publicly available tool—DEPICT—that can address this need by performing integrative analysis, thereby generating novel, testable hypotheses from genetic association studies across a wide spectrum of traits and diseases. Data and software availability The following sections describe the DEPICT methodology in detail. DEPICT source code and example data are available at https://github.com/DEPICTdevelopers . Ready-to-use software is available at www.broadinstitute.org/depict . Definition of associated loci From the set of associated SNPs at a particular threshold (such as genome-wide significance, P <5 × 10 −8 ), we generated independent ‘lead SNPs’ by retaining the most significant SNP from each set of SNPs that are in LD (pairwise r 2 >0.1) and/or in proximity (physical distance of <1 Mb). We computed pairwise LD coefficients based on the imputation panel used in the GWAS, either HapMap Project release 2 and 3 CEU genotype data [27] or 1000 Genomes Project Phase 1 CEU, GBR and TSI genotype data [28] . We defined positions in the human genome according to genome build GRCh37. Next, we created lists of genes at associated loci by mapping genes to loci if they resided within, or were overlapping with, boundaries defined by the most distal SNPs in either direction with LD r 2 >0.5 to the given lead SNP (see Supplementary Note 1 for justification of this locus definition). If no genes were within the locus defined by r 2 >0.5, the gene nearest to the given lead SNP was included. Loci with overlapping genes were then merged. Due to the extended LD in the major histocompatibility complex region and the resulting challenges in delineating associated loci, genes within base pairs 25,000,000–35,000,000 on chromosome 6 were excluded. DEPICT takes as input a set of independent, associated SNPs and automates all other steps outlined here. Gene sets used in DEPICT DEPICT is based on a large number of predefined gene sets from diverse databases and data types ( Supplementary Data 1 ). Gene ontology [15] , Kyoto encyclopedia of genes and genomes [14] and REACTOME [16] gene sets were mapped to Ensembl database identifiers. Molecular pathways were constructed based on experimentally derived high-confidence protein–protein interactions from the InWeb database [17] by considering each of the 12,793 genes in the database and annotating direct, high-confidence interaction partners of a given gene as a molecular pathway (including the given gene itself). We defined high-confidence interactions as pairs of gene products with InWeb-specific protein–protein interaction confidence scores above 0.154, a cutoff previously justified [17] . In addition, we constructed 2,473 phenotypic gene sets based on 211,882 phenotype–gene relationships from the Mouse Genetics Initiative [18] . These gene sets were constructed by adding genes to the same gene set if they were related to the same Mouse Genetics Initiative phenotype. From all repositories, we only included gene sets with at least 10 genes and at most 500 genes. Gene function prediction for gene set reconstitution DEPICT performs gene prioritization and gene set enrichment based on predicted gene function and reconstituted gene sets (note that the reconstituted gene sets are a consequence of the gene function prediction). Please refer to Fehrmann et al . [6] (and www.genenetwork.nl ) for a detailed description of the gene function prediction method. The main hypothesis behind the gene function prediction follows a guilt-by-association logic: a gene that is co-regulated with say 20 other genes, which perform a specific function, is likely to exhibit the same function. In Fehrmann et al . [6] , we developed an approach that quantifies co-regulation between pairs of genes based on gene expression data, even in instances where transcriptomic co-regulation is subtle. In Fehrmann et al . [6] , we conducted the following steps to predict functions of genes and construct reconstituted gene sets: 1 We first renormalized 77,840 microarrays from two human, one rat and one mouse Affymetrix gene expression platform downloaded from the Gene Expression Omnibus (GeO) database [29] ( Supplementary Data 13 ). 2 We constructed a probe–probe correlation matrix (using Pearson correlation to compute all pairwise probesets correlations) for each of the four platforms. 3 We performed principal component analysis on each of the four correlation matrices, and used Cronbach’s Alpha and Split-half reliability statistics to retain 777 and 377 eigenvectors (hereafter ‘transcriptional components’ or ‘TCs’; Fehrmann et al . [6] ) from the two human platforms, 677 TCs from the mouse platform and 375 TCs from the rat platform. 4 We mapped all human genes to Ensembl identifiers [30] ; mouse and rat genes were mapped to their human homologues (Ensembl database orthology mapping). The loadings of each gene on each TC are the elements of a gene-TC matrix with 19,997 gene rows (the number of genes covered by the Affymetrix platforms) and 2,206 TC columns. We then used the gene-TC matrix to predict 19,997 genes’ function across the 14,461 functional annotations represented by the predefined gene sets, by doing the following steps: 1 For each gene set, we computed the enrichment on each TC (using z -scores derived from Welch’s t -test to assess whether the TC loadings from genes from the given set significantly deviated from all other genes’ loadings). This resulted in a TC profile for each gene set (a gene set-TC matrix of z -scores with 14,461 gene set rows and 2,206 TC columns). 2 To obtain gene function predictions and reconstituted gene sets, we quantified each gene’s likelihood of being part of a given predefined gene set by correlating the gene’s 2,206 TC loadings (from the gene-TC matrix) with the z -score TC profile of each gene set (from the gene set-TC matrix). To avoid circularity in cases where a particular gene was part of a predefined gene set, we left out that gene from the gene set, recomputed the gene set z -score profiles along all TCs and then computed the correlation of the gene with the gene set. 3 We converted the correlation P values to z -scores to obtain a gene-gene set matrix of z -scores comprising 19,997 gene rows and 14,461 gene sets columns. This matrix is used by DEPICT to perform gene prioritization and gene set enrichment analysis. Null GWAS construction To take sources of confounding into account, DEPICT makes use of precomputed GWAS based on randomly distributed phenotypes to (‘null GWAS’). We computed 200 GWAS based on genome-wide CEU genotype data from the Diabetes Genetics Initiative [31] (DGI) and simulated Gaussian phenotypes (random draws from N (0,1) distribution) with no genetic basis. DEPICT gene prioritization For gene prioritization, DEPICT employs a phenotype- and mechanism-agnostic algorithm, which is predicated on a previously formulated assumption that truly associated genes share functional annotations [1] , [17] , [32] . In other words, genes within associated loci that are functionally similar to genes from other associated loci are the most likely causal candidates. DEPICT prioritizes genes based on three major steps: a scoring step, a bias adjustment step and a FDR estimation step. In the scoring step, the method quantifies the similarity of a given gene to genes from other associated loci by correlating their reconstituted gene set memberships (across all 14,461 gene sets). The bias adjustment step is designed to control inflation in gene scores caused by, for example, gene length (longer genes are more likely to be part of associated GWAS loci) or structure in the underlying expression data. In this step, the method normalizes the given gene’s similarity score based on the distribution of the given gene’s similarity to genes from 1,000 sets of gene-density-matched loci, derived from the 200 pre-permuted null GWAS. In the last step, experiment-wide FDRs are estimated by repeating the scoring and bias adjustment steps 20 times based on top SNPs from precomputed null GWAS. For a given gene (gene x ) that has a prioritization P value y in the actual data, a FDR is calculated by first counting the number of genes having a P value smaller or equal to y across all 20 null runs and dividing this count by the rank of gene x in the actual data. We note that in the version of DEPICT implemented in the studies of anthropometric traits [10] , [12] , [13] , we included a correction for the number of genes at a given locus. Because this correction does not change gene prioritization results markedly (gene set enrichment results and tissue/cell type enrichment results are unchanged), we recommend not using this correction because it imposes an overly conservative correction on genes in relatively gene-poor loci. This correction was not implemented in the version described here. DEPICT reconstituted gene set enrichment The gene set enrichment analysis algorithm comprises the same three steps as employed in gene prioritization: a gene set scoring step, a bias correction step and a FDR estimation step. For a given reconstituted gene set, DEPICT quantifies enrichment by (1) summing the given gene set membership z -scores (entries in the gene-gene set matrix) of all genes within each associated locus and then computing the sum of sums across all loci; (2) repeating step 1 a thousand times based on random loci that are matched by gene density, and using the thousand null z -scores to adjust the real z -score by subtracting their mean, dividing by their s.d. and converting the adjusted z -score to a P value; and (3) repeating steps 1 and 2 twenty times to estimate experiment-wide FDRs similar to the method described above. DEPICT tissue/cell type enrichment analysis DEPICT utilizes 37,427 human Affymetrix HGU133a2.0 platform microarrays (approximately half of the microarrays used to reconstituted gene sets) to assess whether genes in associated loci are highly expressed in any of the 209 Medical Subject Heading (MeSH) tissue and cell type annotations. The tissue/cell type expression matrix was constructed by averaging gene expression levels of microarray samples with the same MeSH annotation [6] . This process included N (0,1) normalizing across all tissue/cell type annotations to remove effects of ubiquitously expressed genes, N (0,1) normalizing the columns of the tissue/cell type expression matrix (to allow enrichment analysis identical to the gene set enrichment analysis framework) and retaining only tissue/cell type annotations covered by at least 10 microarrays. Conceptually, the resulting gene-tissue/cell type expression matrix resembles the gene-gene set matrix, the only difference being that columns represent the relative expression of genes in a given tissue compared with the other tissues, as opposed to the likelihood of membership of a gene in a gene set. Consequently, the tissue/cell type enrichment analysis algorithm is conceptually identical to the gene set enrichment analysis algorithm. Adjusting for confounding sources For a given set of associated loci from the ‘real GWAS’ (the study of interest), DEPICT extracts the same number of independent loci from the 200 precomputed null GWAS. For a given null GWAS, this is accomplished by varying the SNP association P value cutoff until the number of independent top loci is the same as the number of independent loci in the real GWAS. The independent top loci from each null GWAS are then collected into a single pool of loci. During the DEPICT gene prioritization, gene set enrichment and tissue/cell type enrichment analyses, this pool of loci is used to sample 1,000 collections of gene density-matched ‘null loci’ (in each collection there are as many null loci as the number of loci observed in the real GWAS). Null loci within a given collection are not allowed to overlap (in terms of genes). During the DEPICT background correction step, if a locus from the real GWAS is represented by <10 gene-density-matched null loci, DEPICT iteratively includes larger and smaller null loci (to avoid oversampling the same null loci during the 1,000 background runs). We employed different numbers of null GWAS contributing to the pool of null loci, and observed no major differences between using 200, 500 or 900 null GWAS ( Supplementary Note 3 ). Type-1 error rate analyses To compute type-1 error rates for the gene prioritization, gene set enrichment and tissue/cell type enrichment analyses, we first computed 100 DGI null GWAS the same way as describe in the above section. Spearman correlation coefficients were computed based on log 10 transformed P values. We used an alternate approach to estimate type-1 error by replacing the null GWAS with simulated GWAS that have positive signals but no underlying biological basis. We simulated 50,000 individuals using HAPGEN [33] using parameters from the HapMap Project release 3 CEU population. From this, we obtained 1,175,577 genotypes for all autosomes (chromosomes 1–22) and calculated the allele frequency for each SNP using the 50,000 individuals. We then randomly selected 1,000 SNPs to have an effect on the phenotype and assigned effect sizes such that all SNPs jointly explain 45% of the total variance. The effect size for each SNP was calculated as follows, where β is the effect size in s.d. units, σ 2 is the variance explained for each SNP, p is the SNP’s minor allele frequency and δ denotes a random variable with equal probability of being +1 or −1. Once each SNP’s effect size was determined, we calculated the weighted allele score for each individual by summing up the SNP minor allele dosages weighted by their effect size. The weighted allele score was calculated as follows, where N is the number of SNPs ( N =1,000), β i is the effect size of the i th SNP as calculated earlier, SNP i is the dosage of the minor allele for the i th SNP (0,1 or 2) and p i is the minor allele frequency of the i th SNP. The subtraction of 2 β i p i served to adjust the weighted allele score such that its mean was 0. We obtained the final phenotypic z -score by adding a remaining noise term such that the total variance was 1. The z -score was calculated as follows, where N (0, variance_remaining) is a randomly generated number sampled from a Normal ( N) distribution with mean 0 and variance 0.55. This process was repeated 100 times to obtain 100 sets of phenotypic z -scores for each of the 50,000 individuals. We used PLINK [34] to perform GWAS on each set of phenotypes using the 50,000 simulated genotype samples, and then, for each null GWAS, identified the association P -value threshold that resulted in 100 fully independent loci (DEPICT locus definition). Finally, we ran DEPICT with default settings on each of the n =100 sets of input SNPs. Crohn’s disease DEPICT analysis Summary statistics from GWAS-based meta analysis of Crohn’s disease [23] (downloaded from www.ibdgenetics.org ) were used to identify genome-wide significant loci (using PLINK and parameters ‘--clump-kb 1000 --clump-r2 0.01’). As input to DEPICT we used the resulting 63 genome-wide significant ( χ 2 -test P value <5 × 10 −8 ), which were located in 54 fully independent loci based on DEPICT definitions of independence. Human height DEPICT analysis As input we used 697 genome-wide significant human height associations identified in GWAS-based meta analysis [10] (accessible through http://www.broadinstitute.org/collaboration/giant ), which were located in 566 fully independent loci based on DEPICT definitions of independence. Low-density lipoprotein cholesterol DEPICT analysis Summary statistics from GWAS-based meta analysis of LDL [20] (downloaded from www.sph.umich.edu/csg/abecasis/public/lipids2010 ) were used to identify genome-wide significant loci (using PLINK with parameters ‘--clump-kb 1000 --clump-r2 0.01’). As input to DEPICT we used the resulting 67 independent loci, which resulted in 40 fully independent loci used DEPICT definitions of independence. Gene set enrichment benchmark Due to the lack of an unbiased set of gold standard pathways for any complex trait, we compared DEPICT and MAGENTA [22] by counting the number of statistically significant gene sets predicted based on Crohn’s disease, height and LDL loci. Prior to the benchmark, we estimated the type-1 error rate of both methods by running them with summary statistics from 100 null GWAS constructed based on simulated Gaussian phenotypes with no genetic basis, and HapMap Project release 2 imputed DGI Consortium genotype data ( Supplementary Figs 1 and 3 ). For the null analyses, the top 200 independent loci from each null GWAS were used as input, whereas genome-wide significant loci were used as input in the Crohn’s disease, height and LDL analyses. All MAGENTA runs were based on the complete set of summary statistics. We restricted the comparison to a list of 1,280 gene sets (gene ontology terms, Kyoto encyclopedia of genes and genomes and REACTOME pathways) with overlapping identifiers between both methods. DEPICT was run on reconstituted gene sets. MAGENTA was run with default settings and both methods excluded the major histocompatibility complex region. The non-probabilistic, binary (yes/no) version of the reconstituted gene sets used in one of the MAGENTA comparisons were constructed by applying a threshold on the gene scores for a given reconstituted gene set (all genes above a permutation-based cutoff were considered part of the given reconstituted gene sets, as reported in ref. 6 ). Entries with ‘NA’ in columns ‘DEPICT with predefined gene sets P ’ and ‘DEPICT with predefined gene sets FDR’ in Supplementary Data 4–6 marked predefined gene sets for which enrichment could not be computed in the DEPICT analysis based on predefined gene sets. Gene prioritization benchmark We ran each method (DEPICT and GRAIL [1] ) using their default settings on all genome-wide significant Crohn’s disease [23] , height [10] and LDL [20] associations. To evaluate the methods’ performance on the same set of positive genes (genes that are highly likely to be causal to the phenotype) and negative genes (genes that are unlikely to be causal), we limited the comparison to loci at which there was at least one positive gene present across both methods, and discarded any genes at these benchmark loci that were not considered by each method. For the Crohn’s disease comparison, we used as positives 31 genes that were transcriptionally regulated in whole blood [24] by a genome-wide significant Crohn’s disease association or a SNP in high LD ( r 2 >0.7) with a genome-wide significant SNP. For the height comparison, we used as positives a set of 44 genes that were within genome-wide significant height-associated loci and differentially expressed in rodent growth plate expression studies; we have previously shown that the rodent gene expression data are enriched for genes in height-associated loci [25] ( Supplementary Table 2 in Lango Allen et al . [19] ). For the LDL comparison, we used as positives a set of seven genes with reported Mendelian mutations proposed to cause lipid-related traits [20] . For all three benchmarks, we removed negative genes that had a missense variant in strong LD ( r 2 >0.7) with an associated SNP; for the height and LDL benchmarks, we removed negative genes that were transcriptionally regulated [24] by a SNP in strong LD ( r 2 >0.7) with an associated SNP; in the height benchmark, we removed negative genes that were differentially expressed in rodent growth plates versus other tissues, spatially regulated across different growth plate zones (hypertrophic versus proliferating, and proliferative versus resting) or temporally regulated in growth plates between week 12 and week 3 at nominal significance in reference [25] , and genes that were reported in the high-confidence list in ref. 19 . After these steps, we were able to use 42 negative genes across 18 loci as Crohn’s disease benchmarks and 37 negative genes across 43 loci as height benchmarks. There were no negative genes among the seven LDL benchmark loci. Positive and negatives genes, are listed in Supplementary Data 7–9 . Precision (the fraction of positive genes among all prioritized genes at a given P -value threshold) and recall (the fraction of correctly classified positive genes at a given P -value threshold also referred to as sensitivity) estimates were used to measures accuracy and summarized using the F-measure, which incorporates the ability to recall positive genes with a high precision into a single measure. (Maximum precision implies no false positives, whereas maximum recall implies no false negatives.) To measure the ability to discriminate positive and negative genes at a relative scale, we also computed ROC AUC estimates. To avoid circularity, the growth plate data [25] and the eQTL data [24] were not part of the data used by any of the three methods tested. The R software [35] and the ROCR R library [36] were used to construct the precision recall and ROC curves and the AUC estimates. Prioritizing genes outside genome-wide significant loci To enable prioritization of genes below the genome-wide significance threshold, we scored each gene outside the genome-wide significant loci with respect to its similarity to genes within associated loci. For a given gene outside genome-wide significant loci, we (1) correlated (Pearson) its predicted functions across all 14,461 gene sets to every gene in each of the trait-associated loci, (2) kept the lowest correlation P value from each genome-wide significant locus, (3) converted the P values to z -scores and (4) summed the z -scores and converted the sum back to a P value (alternative hypothesis: gene functionally related to genes in trait-associated loci). We computed FDRs, by redoing steps 1–4 based loci from null GWAS. Using FDR <0.05 as the threshold, we identified 3,022, 5,916 and 1,901 related genes for Crohn’s disease, height and LDL. For each of the three traits, we then calculated genomic inflation factors for SNP P values in the functionally related genes and for SNP P values in the same number of genes exhibiting the highest (non-significant) FDRs. We added 50 kb flanking loci to gene boundaries (defined by the boundaries of the most extreme transcripts) and required genes to be at least 1 Mb away from the nearest genome-wide significant locus. GWAS catalog analysis The GWAS Catalog [26] was downloaded from www.genome.gov/gwastudies/ (download date: 02 January 2014) and 61 phenotypes with at least 10 fully independent regions (DEPICT definitions) based on genome-wide associations were retained. Hierarchical clustering implemented in the R software method ‘hclust’ was run with default settings (method=‘complete-linkage’, dist=‘euclidean’). The DEPICT locus definitions for all GWAS catalog traits can be downloaded from www.broadinstitute.org/mpg/depict . Overlap of gene sets and visualization A previous version of DEPICT used in analyses of anthropometric traits [10] , [12] , [13] computed gene set overlap by imposing a threshold on which genes belong to a given reconstituted gene set and then used the Jaccard index to compute pairwise overlaps. Overlapping reconstituted gene sets were grouped as pathway families. Here, we instead computed the pairwise Pearson correlation between all reconstituted gene sets and then used the Affinity Propagation method [37] to group similar reconstituted gene sets. We named each cluster (‘meta gene set’) by the name of the representative gene set automatically identified by the Affinity Propagation method (for examples, see the top 10 gene set enrichment meta gene sets for Crohn’s disease, height and LDL in Supplementary Data 14–16 ). The R software [35] and a R version of the Affinity Propagation method [38] was used setting the parameters ‘maxits’ to 10,000 and ‘convits’ to 1,000 to ensure conversion when thousands of reconstituted gene sets needed to be clustered. We visualized the overlap between pathway families pathways using Cytoscape [39] . How to cite this article: Pers, T. H. et al . Biological interpretation of genome-wide association studies using predicted gene functions. Nat. Commun. 6:5890 doi: 10.1038/ncomms6890 (2015).